Epistasis between adults and larvae underlies caste fate and fitness in a clonal ant In social species, the phenotype and fitness of an individual depend in part on the genotype of its social partners. However, how these indirect genetic effects affect genotype fitness in competitive situations is poorly understood in animal societies. We therefore studied phenotypic plasticity and fitness of two clones of the ant Cerapachys biroi in monoclonal and chimeric colonies. Here we show that, while clone B has lower fitness in isolation, surprisingly, it consistently outcompetes clone A in chimeras. The reason is that, in chimeras, clone B produces more individuals specializing in reproduction rather than cooperative tasks, behaving like a facultative social parasite. A cross-fostering experiment shows that the proportion of these individuals depends on intergenomic epistasis between larvae and nursing adults, explaining the flexible allocation strategy of clone B. Our results suggest that intergenomic epistasis can be the proximate mechanism for social parasitism in ants, revealing striking analogies between social insects and social microbes. In social organisms, individual phenotypes are influenced by the social environment. For example, social interactions between parents and offspring, sexual partners, or among siblings, can affect the development or behaviour of focal individuals [1] , [2] , [3] , [4] , [5] , [6] , [7] , [8] , [9] . Social insects, like ants and honeybees, often show extreme phenotypic plasticity at the individual level, with queens and workers differing strikingly in morphology, reproductive physiology, longevity and behaviour. While it has recently been shown that an individual’s genotype, and even interactions between the maternal and the paternal halves of the genome, can have strong effects on its developmental trajectory (that is, direct genetic effects) [10] , [11] , [12] , [13] , it is generally believed that in most social insects the caste fate of individuals depends largely on maternal effects [14] and the rearing environment experienced during development [15] , [16] , [17] , [18] . One important component of the rearing environment are the adult workers that care for the larvae, giving rise to sib-social effects on caste fate. If maternal effects or sib-social effects have a genetic basis, that is, depend on the genotype of the mother or workers, respectively, larval development is subject to indirect genetic effects [15] , [16] , [17] , [18] . Finally, direct and indirect genetic effects need not be additive, that is, there can be interaction effects, for example, between the genotypes of the larvae and the genotypes of the workers that raise them [15] , [16] , [17] , [18] . These intergenomic interaction effects, or intergenomic epistasis, are analogous to physiological epistasis within a genome, where the phenotypic effect of the genotype at a given locus depends on the genotypes at other loci within the same genome [16] . In the last few years, cross-fostering experiments between different honey bee strains and subspecies [19] , [20] , [21] , [22] and Temnothorax ant species [15] , [16] have demonstrated that in social Hymenoptera both individual and colony-level phenotypes are influenced by indirect genetic effects and intergenomic epistasis between larvae and workers. However, despite their importance for development and colony organization, the effects of indirect genetic effects and intergenomic epistasis on genotype fitness in competitive situations and associated social evolutionary dynamics have only rarely been studied empirically in social insects. We therefore decided to use the female parthenogenetic (thelytokous) ant Cerapachys biroi to study the relative importance of direct and indirect genetic effects, as well as intergenomic epistasis on phenotypic plasticity and genotype fitness in uniform and mixed social groups. Furthermore, it has been suggested that thelytokous parthenogenesis in social insects might provide an evolutionary route to social parasitism [23] . For example, thelytokous Cape honey bees parasitize a different honey bee subspecies [24] , and in the thelytokous Japanese queenless ant Pristomyrmex punctatus , genetically distinct cheater lineages spread horizontally between host colonies [25] . While socially parasitic lineages have not been reported in C. biroi , we conjectured that a better understanding of indirect genetic effects and the intergenomic epistatic interactions between different genotypes would also have the potential to shed new light on the evolution of social parasitism and the underlying proximate mechanisms. Cerapachys biroi is unusual among social Hymenoptera in that queens are absent, and colonies consist entirely of totipotent workers that reproduce via thelytokous parthenogenesis [26] , [27] , [28] . As a consequence, colonies are composed of individuals that are genetically almost identical, and this applies even to different colonies from the same clonal lineage [27] , [28] . Because different clonal genotypes can be mixed in experimental colonies, this allows us to precisely control and replicate the genetic composition of social groups. All individuals in a C. biroi colony reproduce, at least during the first months of their lives, and individuals are synchronized in their reproduction. Reproduction occurs in stereotypical colony cycles, and a new cohort of workers emerges synchronously approximately every 34 days [29] , [30] , [31] , [32] . Colonies collected in the field usually contain tens to a few hundreds of workers, and in the laboratory, colonies composed of as few as five workers are fully viable. Although the species’ cryptic subterranean lifestyle precludes direct observations in the field, laboratory observations suggest that new colonies are formed by an irregular process in which small colony fragments bud off the mother colony, for example, during colony emigrations or when nest cavities become crowded. Because workers are totipotent and queens are absent, the number of individuals produced by a given genotype during each colony cycle serves as a straightforward measure of genotype fitness. Finally, colonies of C. biroi consist of two worker subcastes that differ in morphology, behaviour and reproductive physiology [29] , [30] , [31] ( Fig. 1 ). High-reproductive individuals (HRIs), which have four to six ovarioles, usually do not forage and lay up to eight eggs per reproductive cycle, and low-reproductive individuals (LRIs), which have two ovarioles, lay at most two eggs per cycle and become sterile foragers at four to five months of age [29] , [30] , [31] . 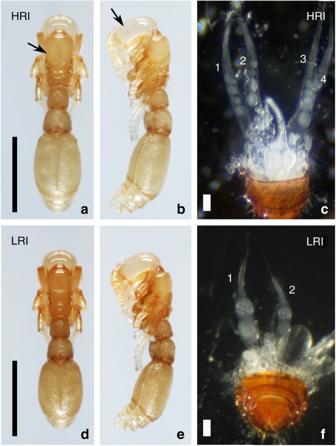Figure 1: The two subcastes ofC. biroi. Dorsal view (a) and lateral view (b) of a HRI pupa, scale bar 1 mm, and ovaries of a HRI (c), scale bar 0.1 mm. Dorsal view (d) and lateral view (e) of a LRI pupa, scale bar 1 mm, and ovaries of a LRI (f), scale bar 0.1 mm. HRIs are slightly larger and have more ovarioles than LRIs. In HRIs, thoracical sutures (arrow ina) are more developed, and they have visible vestigial eyes (arrow inb). Figure 1: The two subcastes of C. biroi . Dorsal view ( a ) and lateral view ( b ) of a HRI pupa, scale bar 1 mm, and ovaries of a HRI ( c ), scale bar 0.1 mm. Dorsal view ( d ) and lateral view ( e ) of a LRI pupa, scale bar 1 mm, and ovaries of a LRI ( f ), scale bar 0.1 mm. HRIs are slightly larger and have more ovarioles than LRIs. In HRIs, thoracical sutures (arrow in a ) are more developed, and they have visible vestigial eyes (arrow in b ). Full size image We conducted two separate experiments: a first experiment in which we studied the fitness of two different clonal lineages (A and B) both in isolation and in chimeric (mixed) colonies (clone-mixing experiment), and a second experiment in which we studied the effect of worker genotype on larval development (cross-fostering experiment). The first experiment shows that clone B consistently outcompetes clone A in chimeric colonies, despite the fact that clone A reproduces faster than B when both are raised in isolation. The likely explanation is that in chimeric colonies, clone B produces essentially all the HRIs, that is, B specializes on reproduction while A specializes on cooperative tasks. The second experiment reveals epistatic interactions between the genotypes of larvae and nursing adults that affect the developmental trajectory of larvae into LRIs versus HRIs. These epistatic interactions probably underlie the shift in caste ratio exhibited by clone B in chimeric colonies. Our results demonstrate that intergenomic epistasis can be a proximate mechanism for social parasitism by regulating the development and fitness of different genotypes in social groups. Clone-mixing experiment We used LRIs from four different laboratory stock colonies belonging to two different clonal lineages (colonies J1 and T5 for clonal lineage A, and colonies O6 and T1 for clonal lineage B; see methods for details) to set up chimeric and monoclonal colonies, which we then propagated for six generations (colony cycles). Each generation of workers was paint marked upon emergence to a posteriori monitor changes in clone ratios and HRI allocation during colony growth. For chimeric colonies, we microsatellite genotyped all HRIs produced throughout the experiment (533 individuals), as well as a subset of LRIs at generations one, two and six, to assign them to clonal lineages (224, 344 and 597 individuals, respectively). We also genotyped all the HRIs produced in monoclonal colonies (180 individuals) to assign them to their respective source colony. In total, we genotyped 1,878 individuals. After six generations, monoclonal A colonies ( n =5) were larger than monoclonal B ( n =8) and chimeric ( n =20) colonies (Kruskal–Wallis test, χ 2 =8.2324, Df=2, P =0.016; post hoc pairwise comparison after Bonferroni correction, α=0.016, both P <0.001; Fig. 2a ), showing that, under our experimental conditions, genotype A has a higher fitness than genotype B in isolation. B and chimeric colonies did not differ significantly in size ( post hoc pairwise comparison after Bonferroni correction, α=0.016, P =0.9). On the basis of these results, we expected that genotype A would outcompete B in chimeras. During the first generation, clone A indeed produced more offspring than clone B, but no differences were found at generation two (generalized linear mixed model, GLMM, respectively, χ 2 =6.3792, Df=1, P =0.01, and χ 2 =0.6812, Df=1, P =0.4; n =20 chimeric colonies; Fig. 2b ). By the sixth generation, however, significantly more B than A individuals were produced (GLMM, χ 2 =84.609, Df=1, P <0.0001; n =20 chimeric colonies; Fig. 2b ). Moreover, while in clone A the HRI proportion did not change significantly between monoclonal and chimeric colonies (GLMM, χ 2 =13.371, Df=2, overall comparison, P <0.0001; post hoc pairwise comparison after Bonferroni correction, α=0.008, P =0.04; n =120 and n =30 observations in chimeric and monoclonal colonies across six generations, respectively), the HRI proportion produced by clone B was significantly higher in chimeras (GLMM, χ 2 =13.371, Df=2, overall comparison, P <0.0001; post hoc pairwise comparison after Bonferroni correction, α=0.008, P =0.002; n =120 and n =48 observations in chimeric and monoclonal colonies across six generations, respectively). As a result, almost all HRIs in chimeras (98%) were produced by clone B, which explains why B outcompeted A, that is, had a higher fitness than A in chimeras. 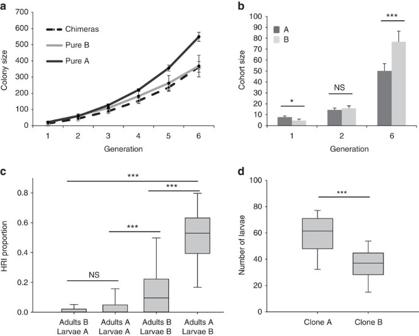Figure 2: Results of the cross-fostering and clone-mixing experiments. (a) Average colony size in monoclonal and chimeric colonies over six generations (mean±s.e.m.;n=20 chimeric colonies,n=5 pure A colonies,n=8 pure B colonies). (b) Number of individuals produced by each clone at generations one, two and six in chimeric colonies (mean±s.e.m.;n=20 colonies). (c) Box-and-whisker plots showing median (horizontal line), interquartile range (box) and maximum/minimum range (whiskers) of the HRI proportions across the four adult-larva combinations in the cross-fostering experiment (GLMM, effect of the larval genotype: χ2=36.179; effect of the treatment: χ2=16.299;n=86 colonies; *P<0.05; **P<0.01; ***P<0.001; NS, not significant). (d) Box-and-whisker plots showing median (horizontal line), interquartile range (box) and maximum/minimum range (whiskers) of the number of larvae produced by each clone in isolation before cross-fostering (GLMM, χ2=53.413, Df=1;n=86 colonies; ***P<0.001). Figure 2: Results of the cross-fostering and clone-mixing experiments. ( a ) Average colony size in monoclonal and chimeric colonies over six generations (mean±s.e.m. ; n =20 chimeric colonies, n =5 pure A colonies, n =8 pure B colonies). ( b ) Number of individuals produced by each clone at generations one, two and six in chimeric colonies (mean±s.e.m. ; n =20 colonies). ( c ) Box-and-whisker plots showing median (horizontal line), interquartile range (box) and maximum/minimum range (whiskers) of the HRI proportions across the four adult-larva combinations in the cross-fostering experiment (GLMM, effect of the larval genotype: χ 2 =36.179; effect of the treatment: χ 2 =16.299; n =86 colonies; * P <0.05; ** P <0.01; *** P <0.001; NS, not significant). ( d ) Box-and-whisker plots showing median (horizontal line), interquartile range (box) and maximum/minimum range (whiskers) of the number of larvae produced by each clone in isolation before cross-fostering (GLMM, χ 2 =53.413, Df=1; n =86 colonies; *** P <0.001). Full size image We then analysed the behaviour of individuals from each separate stock colony within the experiment, to see whether there were differences in HRI production between different stock colonies, both in monoclonal and chimeric experimental colonies. For this step, we used a model that assessed the effect of source colony on HRI production, rather than the effect of clonal lineage (details are given in the Methods section). As expected, we found significant overall differences in HRI production among source colonies in our sample of 33 experimentally mixed colonies (GLM, χ 2 =1445.5, P <0.001). Interestingly, the ratio between source colonies among HRIs deviated from 1:1 not only in the 20 chimeric mixes but also in the eight monoclonal mixes of clone B, whereas no significant deviation was found in the five monoclonal mixes of clone A (GLM with Bonferroni correction, α=0.012, all P <0.001 except for monoclonal mixes of clone A P =0.25. Average HRI proportion in chimeric mixes: colony T5 0.02±0.035 (s.d. ), n =8 observations versus colony T1 0.97±0.035, n =8 observations; colony J1 0.03±0.05, n =12 observations versus colony O6 0.96±0.05, n =12 observations. Average HRI proportions in monoclonal mixes: colony J1 0.66±0.26, n =5 observations versus colony T5 0.33±0.26, n =5 observations; colony T1 0.8±0.02, n =8 observations versus colony O6 0.19±0.18, n =8 observations). Cross-fostering experiment As lineage B changed its HRI production in a context-dependent way, we suspected that this could be due to social influences on larval differentiation, that is, that nursing adults influence larval fate. In other words, we hypothesized that developmental trajectories in C. biroi depend not only on direct genetic effects (that is, larval genotypes) but also on indirect genetic effects (that is, adult genotypes), and possibly interaction effects between larval and adult genotypes. We therefore assessed the propensity of larvae to develop into HRIs when raised by workers of their own or the other clonal lineage. Overall, we found significant effects of the genotype of the larvae, of the treatment (being raised by adults of the same or the other clone) and of the interaction between these two factors (GLMM, respectively: χ 2 =36.179, Df=1, χ 2 =16.299, Df=1 and χ 2 =20.070, Df=1, all P <0.0001; n =86 colonies; large effect size for all factors, respectively: Cohen’s d [33] , [34] 1.68±1.04 (95%CI), 0.74±1.04 (95%CI) and 0.58±1.04 (95%CI)). When raised by clone-mates, B larvae showed a higher tendency to develop into HRIs than A larvae (on average 16.3±16.5% (s.d.) versus 3.4±5.6%, GLMM, χ 2 =14.268, Bonferroni correction, α=0.008, P =0.0001; n =21 colonies each for A and B; Fig. 2c ). While A larvae did not significantly change their HRI differentiation rate when raised by B workers (on average 1.42±3.11%, GLMM, χ 2 =2.5367, Bonferroni correction, α=0.008, P =0.1; n =21 colonies of A larvae raised by A workers and n =22 colonies of A larvae raised by B workers; medium effect size: Cohen’s d=0.43±0.6 (95%CI); Fig. 2c ), B larvae showed a markedly increased propensity to develop into HRIs when raised by A workers (on average 51.7±21%, GLMM, χ 2 =34.98, Bonferroni correction, α=0.008, P <0.0001; n =21 colonies of B larvae raised by B workers and n =22 colonies of B larvae raised by A workers; large effect size: Cohen’s d=1.9±0.7; Fig. 2c ). Possibly due to cannibalism between larvae, overall larval mortality was high (37.5±14.6% (s.d. ); n =86 colonies) but was not influenced by the genotype of the larvae, by the treatment, or by the interaction between these two factors (GLMM, respectively: χ 2 =2.9276, P =0.087; χ 2 =1.8320, P =0.17; χ 2 =1.8596, P =0.17; n =86 colonies). Before cross-fostering, larvae produced by each experimental colony were counted to evaluate the fertility of each clonal lineage. Lineage A produced significantly more larvae than B (GLMM, χ 2 =53.413, Df=1, P <0.0001; n =43 colonies each for A and B; Fig. 2d ), confirming the higher fertility observed in the previous experiment. As the results from the clone-mixing experiment (see previous section) showed that source colony T1 consistently produced more HRIs than source colony O6 when the two were mixed in monoclonal experimental colonies, we tested whether a similar source colony-specific effect was also evident in our cross-fostering experiment. Compared with the clone-mixing experiment, the cross-fostering experiment was conducted over a single generation, allowing us to more precisely standardize group size, group demography and food quantity throughout the entire experiment (see Methods section). As expected based on our analysis at the clone level, we found significant overall differences in the proportion of larvae that developed into HRIs across the different combinations of adults and larvae from different source colonies (GLM, source colony of adults nested within source colony of larvae, χ 2 =66.276, P <0.001; n =86 colonies; Fig. 3a ; GLM, source colony of larvae nested within source colony of adults, χ 2 =221.99, P <0.001; Fig. 3b ). Larvae of clone B (stock colonies O6 and T1) always developed more frequently into HRIs when raised by adults from either of the two clone A stock colonies, although not all individual pairwise comparisons were statistically significant (GLM, post hoc pairwise comparisons after Bonferroni correction, α=0.008; details and sample sizes are given in Fig. 3a, b ). Although larvae of stock colony T5 (clone A) did not show significant differences in HRI differentiation according to the source colony of the nursing adults (GLM, post hoc pairwise comparisons after Bonferroni correction, α=0.008, all P >0.19; details and sample sizes are given in Fig. 3a ), larvae of stock colony J1 (clone A) developed more readily into HRIs when raised by adults from their own stock colony than when raised by adults from either of the clone B stock colonies (GLM, post hoc pairwise comparisons after Bonferroni correction, α=0.008, both P <0.006; details and sample sizes are given in Fig. 3a ). 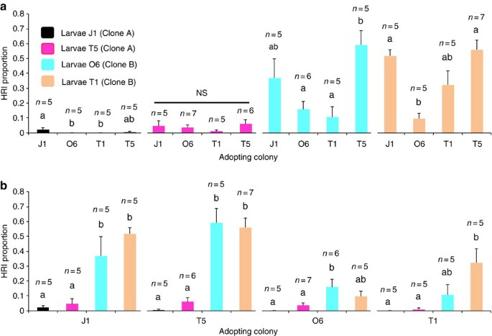Figure 3: Source colony-specific results from the cross-fostering experiment. (a) Bars illustrating the HRI proportions across the sixteen colony-specific adult-larva combinations, with statistical comparisons given according to larval genotype (GLM, χ2=66.276; columns and bars represent average and standard error, respectively; letters a and b indicate statistical significance with α=0.008 after Bonferroni correction; sample sizes are given as the number of colonies above each bar). (b) Same as in (a), but comparisons are given according to adult genotype (GLM, χ2=221.99; columns and bars represent average and standard error, respectively; letters a and b indicate statistical significance with α=0.008 after Bonferroni correction; sample sizes are given as the number of colonies above each bar). Figure 3: Source colony-specific results from the cross-fostering experiment. ( a ) Bars illustrating the HRI proportions across the sixteen colony-specific adult-larva combinations, with statistical comparisons given according to larval genotype (GLM, χ 2 =66.276; columns and bars represent average and standard error, respectively; letters a and b indicate statistical significance with α=0.008 after Bonferroni correction; sample sizes are given as the number of colonies above each bar). ( b ) Same as in ( a ), but comparisons are given according to adult genotype (GLM, χ 2 =221.99; columns and bars represent average and standard error, respectively; letters a and b indicate statistical significance with α=0.008 after Bonferroni correction; sample sizes are given as the number of colonies above each bar). Full size image We have shown that larval caste fate in C. biroi depends on indirect genetic effects from nurse workers, as well as intergenomic epistatic interactions between larvae and nurse workers, both of which in turn affect the outcome of competitive interactions between clones in chimeric colonies. A simple model that can account for our findings is that larvae of different genotypes have different response thresholds to worker cues that inhibit (or promote) HRI development, and adults of different genotypes inhibit (or promote) HRI development at different intensities ( Fig. 4 ). In particular, lineage B larvae have a low HRI differentiation threshold, but B adults exert a strong inhibition that prevents larvae from developing into HRIs. On the other hand, A larvae have a high threshold to develop into HRIs, and A adults display a lower level of inhibition. According to this interpretation, B larvae were only weakly inhibited when raised by A adults in the cross-fostering experiment, which markedly increased their HRI differentiation rate ( Fig. 2c ). The HRI differentiation rate of clone A was already low in control colonies and decreased even further when cross-fostered in B colonies ( Fig. 2c ). However, this decrease was not statistically significant, possibly due to the medium effect size of the treatment for clone A. This interpretation is in accordance with similar genetic effects on caste development thresholds and worker provisioning that have previously been described [18] , [20] , [22] , [31] , [35] , [36] , [37] , [38] . Despite the fact that stock colony T1 consistently produced more HRIs than stock colony O6 when the two were mixed in monoclonal B colonies (that is, similar to the effect observed in chimeric colonies), stock colony O6 always produced more HRIs than its partner colony in chimeric colonies, confirming that our finding that clone B outcompetes clone A in chimeric colonies is not exclusively due to the properties of stock colony T1. Furthermore, our cross-fostering experiment detected no differences between colonies T1 and O6 across experimental treatments ( Fig. 3a, b ), implying that the differences between the two stock colonies detected in our clone-mixing experiment are small compared with differences between clonal lineages. 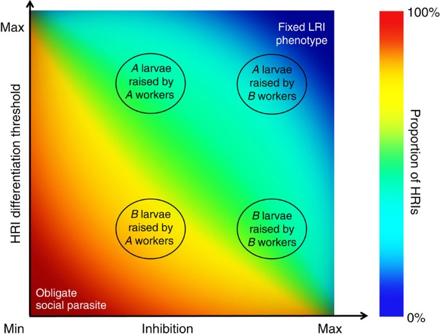Figure 4: Threshold model for caste determination inC. biroi. The proportion of individuals developing into high-reproductive individuals (HRIs) depends on the propensity of larvae to develop as HRIs (‘HRI differentiation threshold’) and on the level of inhibition by adult ants (‘Inhibition’). We hypothesize that the reproductive strategies of differentC. biroiclones are distributed along a continuum, which includes the strategies of clones A and B. The proportion of HRIs raised shifts when larvae are cross-fostered between clones. Phenotypic plasticity is lost at the extremes of the continuum, and only one caste is produced (either LRIs or HRIs). Figure 4: Threshold model for caste determination in C. biroi . The proportion of individuals developing into high-reproductive individuals (HRIs) depends on the propensity of larvae to develop as HRIs (‘HRI differentiation threshold’) and on the level of inhibition by adult ants (‘Inhibition’). We hypothesize that the reproductive strategies of different C. biroi clones are distributed along a continuum, which includes the strategies of clones A and B. The proportion of HRIs raised shifts when larvae are cross-fostered between clones. Phenotypic plasticity is lost at the extremes of the continuum, and only one caste is produced (either LRIs or HRIs). Full size image The results obtained in the cross-fostering experiment are in line with the results of the clone-mixing experiment, suggesting that the same epistatic interactions between larval and worker genomes underlie the elevated proportion of B HRIs raised in chimeric colonies. The mix of A and B adults produced an intermediate level of larval inhibition, resulting in an increased proportion of B larvae and a decreased proportion of A larvae developing into HRIs. The lower fitness of genotype B in monoclonal colonies could be a direct consequence of the caste ratio. HRIs usually do not forage and contribute little to cooperative tasks, and colonies with higher proportions of HRIs might therefore be less efficient at raising offspring. This interpretation is in line with findings in the thelytokous ant Pristomyrmex punctatus , in which colonies with a higher proportion of ‘cheaters’, which behave similar to C. biroi HRIs in that they reproduce more but don’t contribute to cooperative tasks, have lower fitness [39] . In C. biroi , the proportion of HRIs differs across different clones, possibly depending on two individual-level traits, the HRI differentiation threshold of larvae and the level of larval fate inhibition by adults. This ultimately gives rise to the different reproductive strategies of the clonal lineages, including A and B ( Fig. 4 ). The optimal strategy, that is, the optimal ‘calibration’ of the epistatic interaction between larval threshold and adult inhibition, will depend on how frequently mixing occurs in a population, as well as on the larval thresholds and levels of HRI inhibition displayed by other clones in the population. Colonies belonging to clones with an A-like strategy would grow and multiply faster, thereby outcompeting clones with a B-like strategy in populations where genotypes do not mix in chimeric colonies. In contrast, there is an evolutionary trade-off between the reproductive optimum in isolation versus chimeras in populations where genotypes mix. In chimeras, clone B increases its reproductive investment and decreases its allocation to cooperative tasks such as foraging, thereby outcompeting clone A. This plasticity is characteristic of a facultative social parasite. It is conceivable that clone-specific reproductive strategies are distributed along a continuum ( Fig. 4 ). At one extreme of this continuum, the HRI differentiation threshold might be extremely high, the LRI phenotype fixed and the subcaste polyphenism lost. Moving towards the other extreme, the HRI differentiation threshold might decrease and the HRI proportion increase, until the HRI phenotype is fixed and the polyphenism is again lost. Because HRIs usually do not forage, social parasitism would then possibly become an obligatory lifestyle. Our results therefore suggest that intergenomic epistatic interactions between different genotypes can be the proximate mechanism underlying social parasitism. While this has not previously been shown in social insects, the same fundamental mechanism underlies social parasitism (or ‘cheating’) in social microbes like the social amoeba Dictyostelium discoideum . When starved, individual cells aggregate to form a fruiting body consisting of a sterile stalk and a capsule with fertile spores. While stalk cells serve to lift the capsule off the ground, the spores disperse to reach a food-rich medium [40] . Similar to the different HRI allocation ratios in C. biroi , different strains of D. discoideum have fixed spore allocation levels in isolation that undergo a partner-dependent shift in chimeras [41] , [42] , [43] , [44] , [45] , [46] , [47] . Also in this case, differentially calibrated strain-specific systems interact via intergenomic epistasis, resulting in altered spore-to-stalk allocation ratios in chimeric partners. For example, if strain one increases the stalk cell allocation of strain two, while its own spore cell allocation increases due to the weaker stalk cell induction by strain two, this eventually results in strain one outcompeting strain two. A similar scenario is found in the myxobacterium Myxococcus xanthus , where some strains produce more spores in chimeras than in pure culture [48] . Epistatic interactions between social partners therefore have strikingly similar effects on individual phenotypes, social organization and fitness across different levels of biological complexity, from micro-organismal aggregations to the societies of eusocial insects. The fact that only two C. biroi clones and two stock colonies from each clone were available for our study currently limits the generality of our verbal model ( Fig. 4 ). It will therefore be important to study additional clones in the future to verify where they fall on the proposed continuum and to investigate whether our simple threshold model adequately describes pairwise interactions. While clones of D. discoideum indeed form close to linear dominance hierarchies when raised in chimeras [49] , interactions between C. biroi clones could be more complex, resulting in non-linear dominance patterns (for example, by involving additional or different factors than the two proposed thresholds). Furthermore, our results suggest that even genetically highly similar colonies from within the same clonal lineage can show subtle differences in caste allocation, possibly because of small allelic differences, uncontrolled transgenerational effects or minor differences in the rearing conditions of stock colonies. Additional experiments will be required to study these possible effects in detail. While the genetic diversity of C. biroi in the invasive range is limited, it seems to be higher in the native range, from which additional genotypes could potentially be obtained [27] . Despite this limitation, it is interesting in this context that one of the extreme conditions along the proposed continuum is indeed found in the above-mentioned clonal ant P. punctatus, where a parasitic clonal lineage spreads horizontally between host colonies. Individuals of this cheater lineage, which like C. biroi HRIs do not forage, have more ovarioles and lay more eggs than average individuals [29] , [30] , [31] , [50] . As mentioned above, a recent study showed that, in mixed colonies, the P. punctatus cheater lineage performs better than host workers, both in terms of survival and reproduction, while its fitness in isolation is greatly reduced [39] . The P. punctatus cheater lineage is an obligate social parasite, that is, it has lost the phenotypic plasticity that would allow it to function in isolation. To complement the proposed experiments with additional C. biroi clones, it would therefore be interesting to also conduct similar clone-mixing and cross-fostering experiments with different P. punctatus clones other than the obligate social parasite and to see whether the spectrum depicted in Figure 4 can be observed. It is currently also unclear to what extent different C. biroi clones mix in natural colonies, that is, to what extent intergenomic epistasis between different clones affects clone fitness in the field. Colonies of C. biroi discriminate against non-nestmates, especially if they belong to different clones [28] . However, non-nestmate discrimination is never perfect, and our results imply that even small mistakes could have major effects, that is, a single clone B individual could, over time, take over a colony of clone A. So far, all field-collected colonies of C. biroi were monoclonal [27] , [28] . However, this does not necessarily imply that genotypes do not mix in nature. In fact, our results imply that chimeric colonies would be transient and therefore difficult to detect. Moreover, given the broad geographic distribution of C. biroi and its elusive lifestyle, only a few populations have been studied in any detail. In particular, all the relevant population genetic data currently come from a single population in the invasive range, where genetic diversity is extremely low [27] , [28] . Because higher genetic diversity seems to prevail in the native range [27] , chimeric colonies might be more frequent. Under an adaptive scenario, the frequency of clone mixing in nature would have to be sufficiently high to offset the reduced fitness of facultative parasitic genotypes in isolation. Alternatively, certain ecological parameters could favour genotypes with a higher HRI proportion. For example, HRIs could resume reproduction after longer periods of quiescence, while LRIs live shorter and become sterile as they age. A higher proportion of HRIs could therefore be advantageous in fluctuating environments. Future population genetic studies should therefore focus on native populations to provide a better understanding of the prevalence of clone mixing under natural conditions. Irrespective of the precise ecology of the study species in nature, our experiments with chimeric colonies under controlled laboratory conditions have identified important intergenomic epistatic effects on phenotypic plasticity. This fundamental mechanism immediately gives rise to a facultative social parasite phenotype whenever clones mix, and is relevant to the biology of social organisms ranging from microbes to ants. Clone-mixing experiment Experimental colonies were established with callow LRIs (clonal lineage A: colonies J1 and T5 (from Java (Indonesia) and Taiwan, respectively); clonal lineage B: colonies O6 and T1 (from Okinawa and Taiwan, respectively); clonal lineages A and B are two multi-locus lineages (MLLs) referred to as MLL1 and MLL4, respectively, in Kronauer et al. [27] ). We used callow individuals to standardize fertility (there could be age-related changes in egg-production) and avoid potential aggression due to different chemical signatures (callow individuals are chemically insignificant and acquire their cuticular hydrocarbon profile during early adult life). We established 20 experimental colonies by mixing individuals from A and B stock colonies (20 individuals each, total colony size n =40; 12 J1xO6 and eight T1xT5). Thirteen colonies were used as controls (eight BxB (T1xO6) and five AxA (J1xT5)). Colonies were fed ad libitum with live pupae of the ant Aphaenogaster senilis during six colony cycles (roughly seven months). Each new cohort of adult individuals was marked at emergence with a dot of enamel paint on the abdomen. Colonies were killed by freezing when the sixth generation of workers emerged. For DNA extractions, we used the protocol described in Kronauer et al. [28] Each genotyped individual was assigned to one or the other clonal lineage on the basis of two characteristic microsatellite loci (we used different combinations of loci ED32S, ETJ3E, D4XW2, D8M16, ER4IH, D8ZOW, ETCR2 and EFOHK [27] ). To assign individuals to stock colonies in monoclonal experimental colonies, we used combinations of microsatellite loci that differed between stock colonies of the same clonal lineage (D71AW and D4XW2 for clone A colonies, and D6CNC and ESOCS for clone B colonies). We used a Generalized Linear Mixed Model (GLMM) with binomial error and logit-link to compare the proportion of HRIs produced by each clonal lineage in chimeric and monoclonal colonies over the six generations combined. The model included the treatment (experimental or control) and the clonal lineage (A or B) as fixed factors, while the original stock colony and the experimental colony were used as random factors. The overall number of individuals produced by each clone in chimeric colonies at generations one, two and six was analysed with GLMMs with Poisson error and log-link, and included the clonal lineage as fixed factor and the combination of stock colonies (T1xT5, J1xO6) as random factor. All HRIs produced by chimeric colonies from generations one to six were genotyped ( n =533). While all the LRIs of generation one could be genotyped due to the small size of cohorts (on average 14±11 (s.d.) individuals per colony; n =20 colonies), we genotyped a subsample of LRIs of generations two and six due to the large size of cohorts (30.3±14.9 and 127.3±49.1 individuals per colony for generations two and six, respectively; both n =20 colonies). We obtained an estimation of the number of LRIs produced by each clone by multiplying the total number of LRIs produced in that generation by the proportion of LRIs produced by each clone among the genotyped LRIs. We used a GLM with quasibinomial error and logit-link to compare the HRI proportions produced by separate stock colonies in all studied pairwise combinations. All statistical analyses were performed with the software R [51] . GLMs and GLMMs were implemented in the R package lme4 (ref. 52) [52] and corrected for overdispersion when the residual deviance of the data exceeded the residual degrees of freedom. Cross-fostering experiment Experimental colonies were established with 50 callow LRIs (one to two weeks old) to exclude effects of age-related changes in fertility. As HRI production depends on the colony-level proportion of fertile individuals [30] , the exclusive use of LRIs minimized fertility-related biases in the HRI proportion of the focal cohorts of larvae. We used individuals from the same four stock colonies used in the clone-mixing experiment (A: colonies J1 and T5; B: colonies O6 and T1), covering all possible pairwise adult-larvae combinations (at least five repetitions each, 86 experimental colonies in total). Experimental pairs of colonies were established simultaneously, so that egg-laying and larval hatching occurred in synchrony and cross-fostering could be performed with larvae at the same developmental stage (recently hatched L1). Colonies were initially fed identical amounts (0.02±0.0006 (s.d.) g; n =86 feeding events) of live pupae of A. senilis and were not fed again until after cross-fostering. Afterwards, colonies were fed ad libitum with live A. senilis pupae until larvae pupated. As larvae inhibit ovary development in C. biroi [31] , no eggs were laid during the development of the focal cohort (the individuals cross-fostered as larvae), excluding the possibility of clone-mixed cohorts of larvae. Just before callow emergence, the HRI/LRI ratio of the focal cohort was calculated by classifying individuals according to the presence of thoracic sutures and vestigial eyes ( Fig. 1 ). We used a GLMM with binomial error and logit-link to compare the proportion of HRIs developing from larvae raised by their own or the other clonal lineage. The genotype of larvae and the treatment (being raised by adults of their own or the other clone) were implemented as two-level fixed factors, while the colony of origin and the adopting colony were used as random factors. We used GLMs with quasibinomial error and logit-link to compare the proportions of larvae that developed into HRIs for each pairwise combination of separate stock colonies. To evaluate differences in larval mortality, we used a GLMM with binomial error and logit-link, including larval genotype and treatment (being raised by adults of their own or the other clone) as fixed factors, and the original stock colony of adults and larvae as random factors. We used a GLMM with Poisson error and log-link including the clonal lineage as fixed factor and the original stock colony as random factor to detect clone-related differences in brood production. All statistical analyses were performed with the software R [51] . GLMMs were implemented in the R package lme4 (ref. 52) [52] and corrected for overdispersion when the residual deviance exceeded the residual degrees of freedom. How to cite this article: Teseo, S. et al. Epistasis between adults and larvae underlies caste fate and fitness in a clonal ant. Nat. Commun. 5:3363 doi: 10.1038/ncomms4363 (2014).